Reduced-dimensionality-induced helimagnetism in iron nanoislands Low-dimensionality in magnetic materials often leads to noncollinear magnetic order, such as a helical spin order and skyrmions, which have received much attention because of envisioned applications in spin transport and in future data storage. Up to now, however, the real-space observation of the noncollinear magnetic order has been limited mostly to systems involving a strong spin–orbit interaction. Here we report a noncollinear magnetic order in individual nanostructures of a prototypical magnetic material, bilayer iron islands on Cu (111). Spin-polarized scanning tunnelling microscopy reveals a magnetic stripe phase with a period of 1.28 nm, which is identified as a one-dimensional helical spin order. Ab initio calculations identify reduced-dimensionality-enhanced long-range antiferromagnetic interactions as the driving force of this spin order. Our findings point at the potential of nanostructured magnets as a new experimental arena of noncollinear magnetic order stabilized in a nanostructure, magnetically decoupled from the substrate. The magnetic order in solid depends on subtle details of the atomic structure and resulting distribution of the exchange interaction, which occasionally result in noncollinear magnetic order (NCMO) [1] , [2] , where the spins are neither parallel nor antiparallel. The details of the spin order in NCMO may result from different contributions, such as competing exchange interaction [3] , [4] , [5] , Ruderman-Kittel-Kasuya-Yosida (RKKY) interaction, spin–orbit interaction (SOI) [6] , [7] , [8] , [9] , quantum fluctuation of antiferromagnetic (AFM) order [10] and Fermi-surface nesting [11] , [12] , [13] , or their mutual interactions. So far, NCMO’s in the bulk [1] , [2] and at surfaces [6] , [7] , [8] , [9] of materials exhibiting strong SOI have been intensively studied. SOI, in conjunction with broken inversion symmetry, induces a Dzyaloshinskii–Moriya interaction [14] , [15] (DMI), which drives the formation of NCMO, provided its magnitude is comparable to the nearest-neighbour (NN) exchange interaction. Another common origin for NCMO involves long-range AFM interactions, which are of comparable size to the short-range ferromagnetic (FM) interaction [16] . This mechanism has been described within the framework of the Heisenberg exchange model [3] , [4] , [5] , where J ij is the exchange coupling between the pair of spins S i and S j at lattice sites i and j, respectively. NCMO in bulk phases of 3 d itinerant magnetic materials under a drastic change of the atomic volume by few ten % has been predicted by theory [11] . However, in special cases, as observed for Fe, a structural transition from bcc (α-Fe) to fcc (γ-Fe) mediates also a change of magnetic order from FM to AFM, respectively. Structure-related changes of magnetic order are promising for inducing NCMO [17] , [18] . The reduced dimensionalities and symmetries of magnetic nanostructures (MNs), supported on a surface are viable to induce novel magnetic states, which deviate from the respective bulk. This is because of the following: (1) lattice mismatch and epitaxial strain; (2) structural relaxation at interfaces; and (3) structural relaxation induced by finite lateral size and broken in-plane symmetry. These aspects lead to non-bulk-like atomic structures, which in turn modify the spin-dependent electronic properties of MN, resulting in a possible driving force towards NCMO. So far, however, only theory has predicted NCMO in substrate-supported MNs [4] , [5] , [19] . Here we report spin-polarized scanning tunnelling microscopy and spectroscopy (SP-STM/S) studies, combined with ab initio spin-density functional calculations, of a helical spin order (spin helix; SH) in bilayer (BL) Fe nanoislands on Cu(111). It has been proposed that an extended BL Fe film on Cu(111) favours fcc stacking (‘Fe-a’ phase) with a prediction of AFM spin ordering [20] . In contrast, BL Fe nanoislands on Cu(111) with a reduced lateral size (<~10 nm) predominantly show an intriguing lattice structure, which favours a bridge-site-stacking of topmost Fe atoms [20] , [21] (‘Fe-b’ phase). Fe is a prototypical example for studying the impact of structural relaxations on the exchange interaction, because of the pronounced interatomic distance dependence of the magnetic ordering [17] , [18] . This is also corroborated by the prediction of an SH in free-standing monolayers (MLs) of bcc-Fe(110) in theory [12] . In view of a change of spin order, driven by subtle structural changes, the Fe/Cu(001) system is a prototypical example for extended Fe layers [22] , [23] , [24] . We exploit that Fe in bridge-site-stacking is stabilized only in nm-small BLr Fe islands on Cu(111), which plays a pivotal role of the formation of the SH reported here. In these respects, together with a negligibly small SOI of Fe and Cu, the Fe-b phase serves as a prototypical test case to study NCMO localized in a nanostructure, which is almost free from substrate-induced magnetic interactions. Spin-dependent differential conductance of Fe nanoislands The SP-STM/S measurements were carried out at a temperature of 10 K and in an external magnetic field normal to the sample surface (see Methods section). 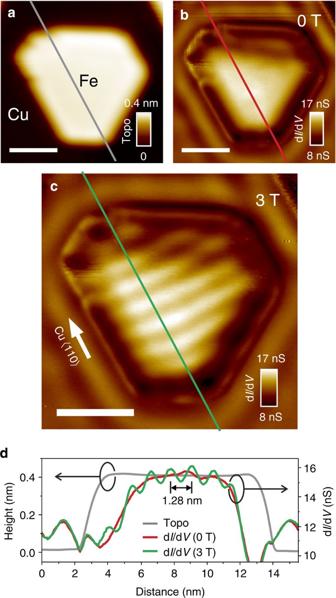Figure 1: Spin-polarized differential conductance map of an Fe island. (a) Constant-current STM image of a bilayer Fe island on Cu(111) (Vb=−0.3 V andISet=3 nA). (b,c) Differential conductance dI/dVimages of the island in (a) at an external magnetic field of 0T (b) and 3T (c;Vb=−0.3 V andISet=3 nA). (d) Profiles along grey, red and green lines ina–c, respectively. Scale bars ina–cindicate 4 nm. Figure 1a shows a constant-current STM (CC-STM) topographic image of a typical Fe island, where the line profile reveals a height of 4 Å (grey curve in Fig. 1d ), indicative of a biatomic layer. The STS spectra identify the island as the structural phase Fe-b [20] , [21] ( Supplementary Fig. 1 ; Supplementary Note 1 ). Figure 1b,c shows the differential conductance d I /d V images measured at 0 and 3 T at 10 K, respectively, of the island shown in Fig. 1a . The differential conductance image at 3 T shows a periodic stripe contrasts with a wavelength of 1.28 nm and a wave vector along the ‹110› direction of the Cu substrate (≈Fe‹110›), which is absent in the differential conductance image at 0 T. The tip shows a non-zero magnetization at 0 T ( Supplementary Fig. 1 ; Supplementary Note 2 ), which indicates that the island does not present a measurable periodic magnetic order at 0 T [25] . Figure 1: Spin-polarized differential conductance map of an Fe island. ( a ) Constant-current STM image of a bilayer Fe island on Cu(111) ( V b =−0.3 V and I Set =3 nA). ( b , c ) Differential conductance d I /d V images of the island in ( a ) at an external magnetic field of 0T ( b ) and 3T ( c ; V b =−0.3 V and I Set =3 nA). ( d ) Profiles along grey, red and green lines in a – c , respectively. Scale bars in a – c indicate 4 nm. 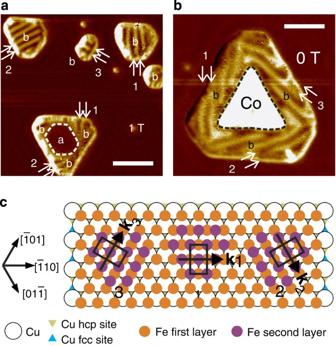Figure 2: Crystallographic symmetry of stripe patterns in Fe islands. (a,b) Differential conductance images of pure Fe islands (a) and an Fe|Co island (b), which show the stripe patterns along three directions denoted by the white arrows with the labels1,2and3. Fe-a and Fe-b regions are indicated by ‘a’ and ‘b’. The white and black dashed lines ina,benclose the Fe-a and Co regions, respectively (Vb=−0.7 V,ISet=3 nA,μ0Hext=1 T fora;Vb=−0.6 V,ISet=3 nA,μ0Hext=0 T forb). (c) Hard sphere model representation of the stacking positions of Fe atoms in the Fe-b phase with respect to the surface lattice of Cu (111) with the crystallographic directions of the Cu (111) surface. The atoms of the first Fe layer are located in the fcc sites of Cu (111), and the atoms of the second Fe layer are at the bridge sites of the first Fe layer21. The bridge-site-stacking allows the formation of three equivalent Fe-b phases, which result from a 120° in-plane rotation. The black rectangles indicate the surface unit cells of the Fe-b phases for three possible in-plane orientations. The black arrows with labelsk1,k2andk3indicate the three wave vectors of the stripe patterns observed in the Fe-b phase, as shown ina,b. Scale bars ina,bindicate 8 and 5 nm, respectively. Full size image Figure 2a,b shows the differential conductance images of pure Fe islands and a Co island in circumferential contact with an Fe BL rim (Fe|Co island) [26] (see also Methods section), respectively, where Co, Fe-a and Fe-b are identified by STS measurements ( Supplementary Fig. 1 ; Supplementary Note 1 ). The stripe patterns are observed also in the Fe-b phases of the Fe rim in Fe|Co islands, with the same wavelength and orientation as in pure Fe-b islands. Interestingly, the stripes show three distinct directions as indicated by the arrows (labels 1, 2 and 3). Correspondingly, the wave vectors of the stripe patterns are oriented along Cu‹110›. These three orientations of the stripe pattern are correlated with the three stacking possibilities of the topmost Fe atoms in the Fe-b phase, as shown in the hard sphere model of Fig. 2c . For all three orientations, we measure a wavelength of the stripe patterns of 1.28±0.01 nm, which is constant, irrespective of island size, shape and bias voltage. A striking aspect is the observation of the stripes at 0 T in the field-dependent differential conductance images of a Fe|Co island ( Fig. 2b ) in contrast to a pure Fe island ( Fig. 1 ). The Co core of the island in Fig. 2b shows a bistable magnetization state with a switching field of 0.75±0.05 T. We propose that the remanent magnetization of the Co core along the out-of-plane direction fixes the Fe spin orientation at the Co–Fe border by exchange coupling [9] , and this ascertains a unique phase of the stripe contrast in each Fe-b region. Figure 2: Crystallographic symmetry of stripe patterns in Fe islands. ( a , b ) Differential conductance images of pure Fe islands ( a ) and an Fe|Co island ( b ), which show the stripe patterns along three directions denoted by the white arrows with the labels 1 , 2 and 3 . Fe-a and Fe-b regions are indicated by ‘a’ and ‘b’. The white and black dashed lines in a , b enclose the Fe-a and Co regions, respectively ( V b =−0.7 V, I Set =3 nA, μ 0 H ext =1 T for a ; V b =−0.6 V, I Set =3 nA, μ 0 H ext =0 T for b ). ( c ) Hard sphere model representation of the stacking positions of Fe atoms in the Fe-b phase with respect to the surface lattice of Cu (111) with the crystallographic directions of the Cu (111) surface. The atoms of the first Fe layer are located in the fcc sites of Cu (111), and the atoms of the second Fe layer are at the bridge sites of the first Fe layer [21] . The bridge-site-stacking allows the formation of three equivalent Fe-b phases, which result from a 120° in-plane rotation. The black rectangles indicate the surface unit cells of the Fe-b phases for three possible in-plane orientations. The black arrows with labels k 1 , k 2 and k 3 indicate the three wave vectors of the stripe patterns observed in the Fe-b phase, as shown in a , b . Scale bars in a , b indicate 8 and 5 nm, respectively. Full size image Magnetic-field-dependent differential conductance of Fe-b A spatially periodic magnetic state could originate from either a collinear spin-density wave [27] , [28] (SDW) or a helical SDW [6] (SH). A collinear SDW is characterized by a periodic change of the magnitude of the spin moments, while the spin orientation is fixed. On the other hand, a SH is composed of spin moments of constant magnitude but with changing orientation. To resolve the origin of the spin ordering in the stripe patterns of the Fe-b phase, we perform SP-STS with a tip, where the direction of the tip magnetization M T can be tuned by the magnetic field [6] . The magnetic characterization of our tip reveals that its magnetization responds to the external magnetic field like a Stoner–Wohlfarth magnet [29] with the magnetic easy axis canted by 55±1° from the sample normal ( Supplementary Fig. 1 ; Supplementary Note 2 ). Therefore, the tip used here is sensitive to both in-plane and out-of-plane components of the sample magnetization at 0 T, while it is sensitive only to the out-of-plane component of the sample magnetization at large field (~±1.5 T). The d I /d V signal in SP-STS depends on m T ˙ m S , where m T and m S are the unit vectors along the directions of tip and sample magnetizations, respectively [25] . Accordingly, the magnetic-field-dependent differential conductance measurement for a collinear SDW will result only in a change of magnitude but not in the phase of the spatial dependence of the d I /d V data. In contrast, the SH will show a field-dependent phase shift of the stripe pattern of the differential conductance signal, since the tip gets more sensitive to the out-of-plane component of the sample magnetization as the magnetic field increases. 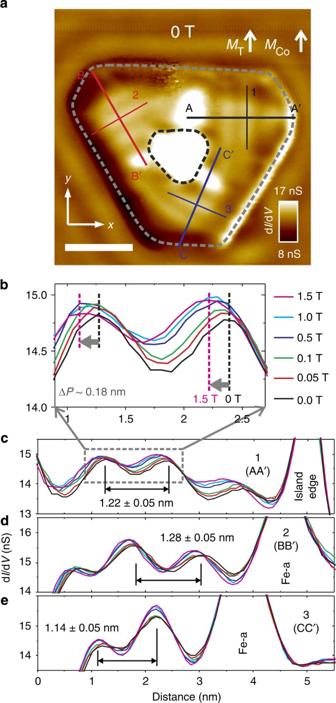Figure 3: Field-dependent differential conductance signals in Fe-b phases. (a) Differential conductance dI/dVmap of an Fe|Co island measured at 0 T, where both magnetizations of tipMTand Co coreMCopoint up (Vb=−0.3 V,ISet=3 nA). The island edges and Co core are indicated by the grey and black dashed lines. The black, red and blue solid lines (arrows) indicate the directions of the stripes (wave vectors of the stripe patterns), corresponding to the Fe-b regions 1, 2 and 3, respectively. (c–e) Field-dependent differential conductance dI/dVprofiles along the arrows1(c),2(d) and3(e) ina, measured with the field sweep from 0–1.5 T. (b) Magnified view of the grey dashed box incand is shown for a clarity of field-dependent peak position shifts inc. The black and purple dotted lines denote the peak positions of the profiles measured at 0 and 1.5 T, respectively. Scale bar inaindicates 4 nm. Figure 3a shows the differential conductance image of an Fe|Co island, measured at 0 T. The Fe-b regions at the three corners of the island show a stripe contrast along three different directions as indicated by the solid lines superposed along the stripes with the labels 1–3. Figure 3c–e shows the field dependences of the differential conductance profiles along the lines AA′, BB′ and CC′ perpendicular to the three directions of the stripe patterns in Fig. 3a , respectively. The wavelengths of the stripe patterns for all three directions, as denoted in Fig. 3c–e , are identical within error margins of ±0.1 nm, and exhibit the same value of 1.28 nm as observed in the pure Fe island ( Fig. 1c,d ). Figure 3b shows a zoom-in of the field dependence of the two peaks in the profiles along the line AA′, as shown within the grey dashed line in Fig. 3c , for clarity. With increasing magnetic field, the positions of maxima and minima move monotonically from right to left, while the distance between the extrema remains constant. A phase shift of Δ P ~0.18 nm is measured upon a change of the magnetic field from 0–1.5 T. This observation rules out a collinear SDW. Rather, the in-field SP-STS identifies a SH as the spin ordering of the stripe contrast in the Fe-b phase. The extrema of stripe patterns at three corners of the island, with increasing field, show different amounts of phase shifts. We perform a quantitative analysis of the phase shift Δ P and its dependence on stripe orientation and field ( Supplementary Fig. 2 ; Supplementary Note 3 ). An excellent agreement between the experiments and simulations ( Supplementary Fig. 3 ; Supplementary Note 4 ) reveals that the field dependences of the phase shifts are determined by a given orientation of the tip magnetization. Figure 3: Field-dependent differential conductance signals in Fe-b phases. ( a ) Differential conductance d I /d V map of an Fe|Co island measured at 0 T, where both magnetizations of tip M T and Co core M Co point up ( V b =−0.3 V, I Set =3 nA). The island edges and Co core are indicated by the grey and black dashed lines. The black, red and blue solid lines (arrows) indicate the directions of the stripes (wave vectors of the stripe patterns), corresponding to the Fe-b regions 1, 2 and 3, respectively. ( c – e ) Field-dependent differential conductance d I /d V profiles along the arrows 1 ( c ), 2 ( d ) and 3 ( e ) in a , measured with the field sweep from 0–1.5 T. ( b ) Magnified view of the grey dashed box in c and is shown for a clarity of field-dependent peak position shifts in c . The black and purple dotted lines denote the peak positions of the profiles measured at 0 and 1.5 T, respectively. Scale bar in a indicates 4 nm. Full size image Theoretical study of SH in BL Fe on Cu(111) The wavelength of the SH (1.28 nm) corresponds to only about five surface lattice constants of Cu along ‹110›. It results in an angle of ≈36° between NN spin moments. This is striking since such a large canting angle gives rise to a dramatic increase in the NN exchange energy. Consequently, another interaction is operative, which compensates this cost of exchange energy. To solve this puzzle, we apply noncollinear spin-density functional theory (see Methods section) to determine the magnetic energy for BL Fe on Cu(111) with the topmost Fe in a bridge position, as illustrated in the inset of Fig. 4a . 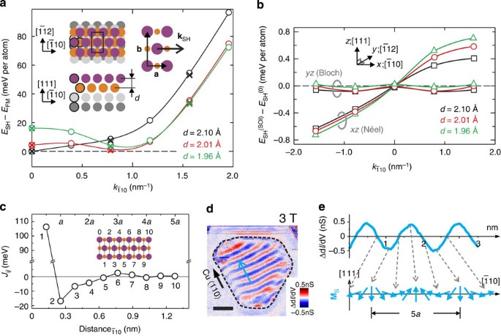Figure 4: Calculated formation energy (ESH−EFM) and magnetic ordering of SH in the Fe-b phase. (a) Circles are the calculated formation energies of SH without SOI, as a function of wave vectorkSHalong the SH direction observed in the experiment at the Fe–Fe interlayer distancesd=2.10, 2.01 and 1.96 Å. The structure of the calculation model, a BL Fe on Cu(111) with topmost Fe in bridge-site-stacking, is depicted by a hard sphere model (top and side views, surface unit cell) in the inset. (aandb) are the surface lattice vectors along theanddirections, respectively. Here the surface lattice constants of BL Fe of an exact epitaxy on Cu(111) (a=2.55 Å andb=4.42 Å) are used. The reference (zero) energy is chosen for the FM stateEFM(kSH=0), which results ind=2.10 Å. Crosses represent the calculated formation energies of SH with SOI, and are superimposed on the curves. (b) Energy difference of the SH structures with () and without () SOI,, atd=2.10, 2.01 and 1.96 Å. The labelsxzandyzindicate the planes of the atomic spin vectors in an SH (thus, Néel- and Bloch-type spin moment arrangements, respectively), where the directionsx,yandzare taken as,and [110], respectively. Note that an asymmetry with respect to theappears in the results forxzcase by an introduction of SOI. (c) Exchange interaction parametersJij, fori=0 andj=1–10 as indicated in the inset, extracted by applying the one-dimensional (alongdirection) effective Heisenberg model toESH−EFMwithd=2.01 Å for the non-relativistic case (red circles) ina,d. Pure magnetic-field-induced variation of the dI/dVsignal ΔdI/dVin the Fe island shown inFig. 1a, extracted by the subtraction of the dI/dVmap at 0 T (Fig. 1b) from that at 3 T (Fig. 1c). The black dashed curve denotes the island edge. The magnetic response ΔdI/dVhere reflects only the position dependence of the out-of-plane component of the sample magnetizationMSsince the tip magnetizationMTis aligned to the direction of the external magnetic field (Supplementary Fig. 1;Supplementary Note 2). Scale bar indicates 3 nm. (e) Position dependence of local magnetization (cyan arrows) is sketched with the ΔdI/dVprofile along the arrow ind. Figure 4a shows the SH formation energy E SH − E FM as a function of the wave vector , at three different Fe–Fe interlayer distances, where d =2.10 Å indicates the FM state of the system ( Supplementary Methods ). First, we calculated the formation energy of a SH state, where the SOI was not taken into account (circles). Interestingly, at reduced interlayer distances—which are expected for the BL Fe on Cu(111)—energy minima (of Δ E ~10 meV per atom) develop. The minima get more pronounced for smaller d . The wave vector at the energy minima corresponds to a SH wavelength of 1.1±0.15 nm, which is in favourable agreement with the experimental observation. Next, we calculate the SH formation energies including SOI and superimpose the results (crosses) in Fig. 4a . The SOI does not lead to any notable contribution to the total SH formation energy. We show the contribution of SOI to the total SH formation energy in Fig. 4b , where and represent the energies calculated with and without SOI, respectively. The size of SOI energy is less than ~0.5 meV per atom at of the energy minima. This is by a factor of order 20 smaller than the energy minima shown in Fig. 4a . To account for a possible impact of in-plane structural relaxation in the Fe-b phase proposed in an earlier report [21] , we also performed the same calculations for free-standing BL Fe systems of a bridge-site interlayer stacking with two different sets of lattice constants ( Supplementary Fig. 4 ; Supplementary Note 5 ). Surprisingly, the effect of a reduced interlayer distance d is more pronounced. The in-plane relaxation even lowers the SH energy minima from those of the unrelaxed structure by ~20 meV per atom ( Supplementary Fig. 4 ; Supplementary Note 6 ). Figure 4: Calculated formation energy ( E SH − E FM ) and magnetic ordering of SH in the Fe-b phase. ( a ) Circles are the calculated formation energies of SH without SOI, as a function of wave vector k SH along the SH direction observed in the experiment at the Fe–Fe interlayer distances d =2.10, 2.01 and 1.96 Å. The structure of the calculation model, a BL Fe on Cu(111) with topmost Fe in bridge-site-stacking, is depicted by a hard sphere model (top and side views, surface unit cell) in the inset. ( a and b ) are the surface lattice vectors along the and directions, respectively. Here the surface lattice constants of BL Fe of an exact epitaxy on Cu(111) ( a =2.55 Å and b =4.42 Å) are used. The reference (zero) energy is chosen for the FM state E FM ( k SH =0), which results in d =2.10 Å. Crosses represent the calculated formation energies of SH with SOI, and are superimposed on the curves. ( b ) Energy difference of the SH structures with ( ) and without ( ) SOI, , at d =2.10, 2.01 and 1.96 Å. The labels xz and yz indicate the planes of the atomic spin vectors in an SH (thus, Néel- and Bloch-type spin moment arrangements, respectively), where the directions x , y and z are taken as , and [110], respectively. Note that an asymmetry with respect to the appears in the results for xz case by an introduction of SOI. ( c ) Exchange interaction parameters J ij , for i =0 and j =1–10 as indicated in the inset, extracted by applying the one-dimensional (along direction) effective Heisenberg model to E SH − E FM with d =2.01 Å for the non-relativistic case (red circles) in a , d . Pure magnetic-field-induced variation of the d I /d V signal Δd I /d V in the Fe island shown in Fig. 1a , extracted by the subtraction of the d I /d V map at 0 T ( Fig. 1b ) from that at 3 T ( Fig. 1c ). The black dashed curve denotes the island edge. The magnetic response Δd I /d V here reflects only the position dependence of the out-of-plane component of the sample magnetization M S since the tip magnetization M T is aligned to the direction of the external magnetic field ( Supplementary Fig. 1 ; Supplementary Note 2 ). Scale bar indicates 3 nm. ( e ) Position dependence of local magnetization (cyan arrows) is sketched with the Δd I /d V profile along the arrow in d . Full size image Our SP-STM/S observations indicate a novel, previously not described, helical spin order stabilized in a single nanostructure, which is magnetically decoupled from the substrate. This is in contrast to previously reported SHs in ultrathin magnetic films on W and Ir [6] , [8] , [9] , where a sizable DMI [14] , [15] , induced by a large SOI at the film–substrate interface, has been identified as the origin of the SH formation. Our ab initio calculations exclude the role of SOI on the formation energy of our SH. The negligible contribution of SOI in the Fe-b system is ascribed to the small spin–orbit coupling strength of the 3 d elements Fe and Cu, which is expected to be an order of magnitude weaker than that of 5 d components [30] (for example, W or Ir). The compilation of the J i,j elucidates the physical origin of SH formation in this system. We extract interatomic exchange interaction parameters J i,j for a SH state in this system by applying one-dimensional effective Heisenberg model to the calculated SH formation energies. Figure 4c shows the interspin distance-dependent J i,j , extracted from the E SH − E FM values of d =2.01 Å (red circles) in Fig. 4a , between i =0th and j =1st to 10th rows along the direction as indicated in the inset. The J 01 is a positive value of ~108 meV, which means that it favours a FM NN spin alignment. On the other hand, the J s from the second to the fifth neighbour ( J 02 – J 05 ) are negative, and this favours AFM spin alignments. These sizable AFM J s of the long-distant neighbours [13] reflect the lowering of the energy by the helical arrangement of the spin moments in Fe-b within the Heisenberg model. Although its magnitude is minute, a quantitative discussion of SOI in this system provides insights into the local magnetic ordering of the SH [12] . An interesting point is that a SH of the spin vectors rotating in the xz plane gives rise to an asymmetry in about . This spin structure contributes a much larger SOI energy with a positive (negative) sign, as compared with a SH rotating in the yz plane, for a positive (negative) wave vector. The asymmetry in SOI with respect to k SH is ascribed to the contribution of the spatially antisymmetric DMI [14] , [15] ( Supplementary Discussion ). The inspection of SOI in this system reveals that a spin rotation in the xz plane with a negative k SH is energetically favoured, giving rise to a Néel-type spin rotation with left-handed chirality, as depicted in Fig. 4e . To understand the absence of magnetic stripe contrast at zero-field in a pure Fe island ( Fig. 1b ), it is instructive to consider the relevant energy scale. The tip shows a non-zero magnetization at 0 T ( Supplementary Fig. 1 ; Supplementary Note 2 ). Thus, we ascribe the absence of zero-field spin-contrast to coherent fluctuation of the spin order in the SH, which are fast on the timescale of STM (several ten seconds). Thus, we speculate that the SH is present at 0 T; however, its phase fluctuates, rendering it invisible to the SP-STM/S. The Zeeman energy E Zee at 3 T amounts to only 0.38 meV per atom ( Supplementary Discussion ). This is smaller by a factor of order 300 (30) than the NN (next NN) exchange energy of the SH in our theoretical prediction. This reveals that our magnetic fields are by far too weak to modify the metric of the SH. However, still, a moderate field is sufficient to stabilize the phase of the SH. This is ascribed to the magnetic field interacting with uncompensated spin moments of SH. The finite lateral size of the island may work as a factor in determining the unique phase of the SH in the following way: a SH length l SH ≠ nλ SH , where n =integer, induces uncompensated net magnetic moment at either end of a SH. This uncompensated moment tends to align its direction parallel to the external magnetic field, providing stabilization of the phase in magnetic fields. In addition, a higher spin state [5] , [31] and larger susceptibility of the spins at the island edge would facilitate this process further. Moreover, the observation of the stripe contrast at 0 T in Fe-b regions of an Fe|Co island excludes the role of the E Zee on the formation of SH. Hence, we neglect the role of E Zee on the field-dependent changes in the differential conductance shown in Fig. 3c–e . The estimation of the magnetic anisotropy (MA) energy E MA of the Fe-b structure, from a hypothetically calculated FM state ( d =2.10 Å; k SH =0), favours a MA along the out-of-plane direction [111] fcc . The energy gain is 0.33 and 0.24 meV per atom as compared with magnetization along two primary in-plane directions and , respectively ( Supplementary Discussion ). The thermal energy E th at our measurement temperature of 10 K is 0.86 meV ( Supplementary Discussion ). All these energy scales are by far too small to form or change the internal spin structure of the observed SH in this study, which is because of orders of magnitude larger J ij . This supports the view that the formation of the SH in Fe-b is driven by a subtle interplay of the exchange interaction acting differently at different spin–spin distances. Thermal energy [32] or zero point energy [33] may drive the fluctuation of the phase of the SH, which results in an averaged-out magnetic signal in SP-STM/S at 0 T. In conclusion, our combined experimental and theoretical studies on the BL Fe nanoisland on Cu (111) reveal a helical spin order in a system, where SOI and magnetic interactions with the substrate are negligible. This spin order is driven by sizable long-distance AFM exchange interactions, which arise from nanosize-driven structural relaxations. The observation of helimagnetism in Fe nanostructures on a light 3 d -element substrate sheds fresh light on the importance of competing exchange interactions on different length scales, arising from the reduced dimensionality of the nanostructures, as a driving force of noncollinear spin states. Our study opens the way for alternative venues to produce noncollinear spin states for potential applications of the MNs. Experiments The experiments were performed in an ultrahigh vacuum (UHV) chamber (base pressure <1 × 10 −11 mbar) equipped with a STM operating at 10 K and a superconducting magnet for magnetic field of up to 7 T, normal to the sample surface. The Cu (111) single crystal substrate (MaTeck GmbH) was cleaned by the repetition of Ar + -sputtering (1 keV, 0.75 μA sample current and 15 min per cycle) and subsequent heating at 700 K for 15 min until defect-free, atomically flat and clean, and large (>200 nm) terraces are observed in STM. We deposit 0.24-ML Co, and then, subsequently, 0.28-ML Fe on the cleaned Cu surface at 300 K in UHV. The sequential deposition leads to the formation of two different types of islands on the Cu substrate; Fe|Co island and isolated Fe island, both are BL high. STM and STS on an Fe|Co island revealed that the distinction between Co and two different Fe structural phases is possible by a difference in apparent heights and pronounced spectroscopic signatures in the differential conductance [26] . In order to obtain magnetic contrast, we used Cr/Co-coated W tips. To obtain a Cr/Co-coated W tip, we deposited 40 atomic layers of Co and 40 atomic layers of Cr subsequently on an electrochemically etched W tip, which was briefly heated in UHV up to 2,400 K for 2 s before the depositions. Then, the Cr/Co-coated W tip was annealed at 600 K for 5 s. We employed a lock-in technique with a modulation bias voltage at a frequency v =4 kHz and of a root-mean square amplitude of 20 mV to detect the tunnel current I ( V ) and the differential conductance d I /d V simultaneously. Point spectroscopy is performed by positioning the tip at the position of STS measurement and before switching the feedback loop off, we stabilize the tip-sample junction at the bias voltage V Stab =0.5 V and the tunnelling current I Stab =1 nA. Theory Density functional calculations were performed based on generalized gradient approximation by using full-potential linearized augmented plane-wave method in which the valence states are treated scalar-relativistically, that is, without SOI, and generalized Bloch theorem is applied for helical spin structures. The SOI was included by the second variational method. Calculations were carried out by: first allowing the interlayer distances in the film to relax by atomic force calculations within the FM state, then the formation energy of the SH state is obtained by varying the Fe–Fe interlayer distance. We extract the exchange interaction parameter J ij for an interatomic row (along direction) by applying the back Fourier transformation of the calculated SH formation energy E SH − E FM with one-dimensional effective Heisenberg model along the direction. More details of the calculation are given in the Supplementary Methods . How to cite this article: Phark, S.-H. et al. Reduced-dimensionality-induced helimagnetism in iron nanoislands. Nat. Commun. 5:5183 doi: 10.1038/ncomms6183 (2014).